Engineering polar discontinuities in honeycomb lattices Unprecedented and fascinating phenomena have been recently observed at oxide interfaces between centrosymmetric cubic materials, where polar discontinuities can give rise to polarization charges and electric fields that drive a metal–insulator transition and the appearance of a two-dimensional electron gas. Lower-dimensional analogues are possible, and honeycomb lattices offer a fertile playground, thanks to their versatility and the extensive ongoing experimental efforts in graphene and related materials. Here we suggest different realistic pathways to engineer polar discontinuities in honeycomb lattices and support these suggestions with extensive first-principles calculations. Several approaches are discussed, based on (i) nanoribbons, where a polar discontinuity against the vacuum emerges, and (ii) functionalizations, where covalent ligands are used to engineer polar discontinuities by selective or total functionalization of the parent systems. All the cases considered have the potential to deliver innovative applications in ultra-thin and flexible solar-energy devices and in micro- and nano-electronics. Combining together different materials rarely results in a simple ‘arithmetic sum’ of their properties. Typically, the composite system displays properties that are not present in its components, giving rise to novel and unexpected behaviour. This is the case for oxide interfaces, which have been recently attracting considerable attention, both experimentally and theoretically [1] , [2] . Among these, a dominant role is played by heterostructures of strontium titanate (SrTiO 3 or STO) and lanthanum aluminate (LaAlO 3 or LAO). Both LAO and STO are insulators; nevertheless, when brought together, a two-dimensional electron gas (2DEG) with high mobility appears at their interface [3] . This 2DEG is host to a rich variety of phenomena, ranging from superconductivity [4] to magnetism [5] (and even the unprecedented combination of the two [6] , [7] ), with many promising device applications. The most intuitive picture to explain the existence of the 2DEG follows from dielectric considerations on the bulk properties of the constituent compounds [8] . LAO and STO have an identical cubic centrosymmetric crystal structure; therefore, classically, the macroscopic polarization of each material should be zero, thanks to inversion symmetry. However, in the framework of the Modern Theory of Polarization [9] , polarization cannot be represented by a single vector, but as a lattice of vectors with the same periodicity of the crystal lattice and satisfying all the symmetries of the crystal. For cubic systems that display inversion symmetry, this condition allows two different polarization lattices, one containing the zero vector and another shifted by half of the cube diagonal. STO belongs to the first class, while LAO to the second, and as a result, a polar discontinuity appears when LAO is epitaxially grown on top of STO and a polarization charge builds up at the interface [8] . This discontinuity creates an electric field inside LAO that can in turn induce a metal–insulator transition with a transfer of free charges from the surface of LAO to the STO/LAO interface [8] , [10] . This transition has been found experimentally to occur at LAO thicknesses of three to four layers [11] , in agreement with theoretical calculations [8] . Such concepts could be extended to lower dimensions, with one-dimensional (1D) channels of free carriers appearing at the boundary between two-dimensional (2D) insulating materials, provided that the ‘bulk’ polarizations of the 2D crystals involved were different. In this respect, non-centrosymmetric honeycomb lattices offer a very promising playground, owing to the quantized and topological nature of their bulk polarization [12] , [13] . A suggestion in this direction has been put forward in ref. 14 , where the authors have considered honeycomb crystals of aluminum nitride, silicon carbide (SiC) and zinc oxide (ZnO). First-principles simulations have confirmed the existence of a polar discontinuity at the interface between two such crystals, with free charges accumulating in 1D channels along the interfaces [14] . In the thermodynamic limit, the linear charge density λ F of free carriers perfectly balances the polarization charge density λ P and it is thus determined solely by the bulk properties of the materials involved and by the orientation of the interface through [15] Here P 1,2 are the bulk polarizations of the parent crystals and is a unit vector normal to the interface and pointing from 1 to 2. Although the suggestion for an analogue in 2D of the LAO/STO heterostructure is very promising, a practical concern hinders the feasibility of the setup suggested in ref. 14 . Indeed, although ZnO and SiC have been synthesized as few-layer hexagonal structures [16] , [17] , they have not been isolated as monolayers, and the realization of in-plane heterostructures seems even more demanding. In this study we outline instead experimentally viable approaches to the realization of polar discontinuities at the interface between honeycomb structures, giving rise to 1D wires of electrons and holes, and opening the possibility of manifold applications. First, we note that vacuum can be interpreted as an insulator with vanishing polarization. Thus, in a nanoribbon made out of any polar lattice, polarization charges will appear as a consequence of the polar discontinuity at its edges (that is, at the interface with vacuum). Second, we argue that covalent functionalizations (for instance, with hydrogen or fluorine) can change the polarization of the parent crystal. Partial functionalization of a 2D sheet thus introduces a discontinuity in the electric polarization at the boundary between functionalized and pristine regions. Alternatively, full functionalization of the recently reported [18] , [19] , [20] , [21] , [22] lateral heterostructures between graphene and boron nitride (BN) can also be pursued. We illustrate in the following all these strategies in more detail, starting from those that are conceptually simpler and highlighting for each the challenge or simplicity of their experimental realization. Last, we support these suggestions with the results of extensive first-principles numerical simulations. Nanoribbons of sp materials As a first suggestion, we consider the case of pristine nanoribbons (see Fig. 1a ) where the discontinuity has to be considered with vacuum. 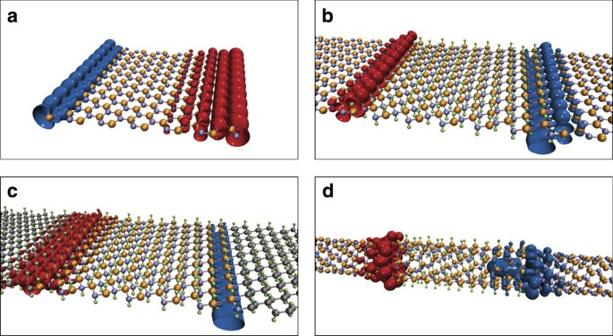Figure 1: Possible realizations of polar discontinuities in honeycomb lattices. (a) Zig-zag nanoribbon from a 2D heteronuclear honeycomb lattice (in this case, boron nitride with unsaturated edges), where the ‘interface’ is with vacuum (i.e., an insulator with vanishing polarization). (b) Selective covalent functionalization (for example, with hydrogen) of a parent honeycomb lattice (here, boron nitride). (c) Full functionalization of a heterostructure of graphene and boron nitride. (d) Selective covalent functionalization of a nanotube. In all panels, the real-space distribution of free-carrier density is plotted in red (blue) for electrons (holes). According to the interface theorem [15] , the polarization charge density is related to the bulk formal polarization [9] , which, for non-centrosymmetric honeycomb crystals, is constrained by symmetry to have quantized values and to point along one of the equivalent armchair directions [12] , [13] , [14] : Figure 1: Possible realizations of polar discontinuities in honeycomb lattices. ( a ) Zig-zag nanoribbon from a 2D heteronuclear honeycomb lattice (in this case, boron nitride with unsaturated edges), where the ‘interface’ is with vacuum (i.e., an insulator with vanishing polarization). ( b ) Selective covalent functionalization (for example, with hydrogen) of a parent honeycomb lattice (here, boron nitride). ( c ) Full functionalization of a heterostructure of graphene and boron nitride. ( d ) Selective covalent functionalization of a nanotube. In all panels, the real-space distribution of free-carrier density is plotted in red (blue) for electrons (holes). Full size image In equation (2), a 1 and a 2 are the primitive lattice vectors (see Fig. 2 ), R is a generic Bravais lattice vector, Σ is the area of a unit cell and m ε{0,1,2}. The value of m can be simply obtained once the ground state of the system is expressed in terms of a set of maximally localized Wannier functions [23] . If desired, standard choices for the gauge vector R in equation (2) can be made by assigning each Wannier function to a given ion according to the crystal termination [24] . 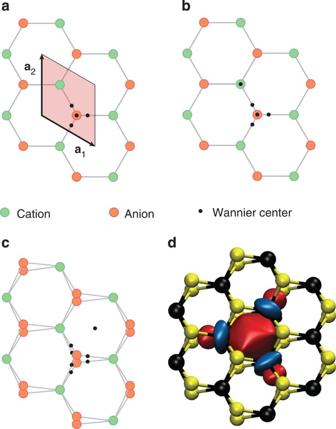Figure 2: Maximally localized Wannier functions in non-centrosymmetric honeycomb lattices. (a) Crystal structure of a typical heteronuclear honeycomb lattice. Each unit cell, identified by two lattice vectorsa1anda2, includes two inequivalent lattice sites, occupied by a cation-like and an anion-like atom, respectively. Inspmaterials, the upper valence bands can be mapped into four doubly degenerate Wannier functions centred around the anion. When the parent crystal is functionalized with hydrogen in a chair configuration the effect is twofold: (i) the effective ionic charge at each lattice site is increased by one unit and (ii) an additional Wannier function has to be included to accommodate the extra electrons. As shown inb, the in-plane projection of the corresponding centre is on top of the cation, while the other four Wannier functions remain localized around the anion, as in panela. (c) Wannier function centres for group VI transition metal dichalcogenides (for example, MoS2, WSe2and so on). Six doubly degenerate Wannier functions are located around the chalcogens, while another one is located in the middle of the hexagonal cell. (d) Isosurface plot for the latter Wannier function in MoS2(Mo atoms in black and S atoms in yellow). Then, the electronic contribution to P can be expressed as a sum over point-like charges located at the Wannier centres ‹ r › j and the total formal polarization reads Figure 2: Maximally localized Wannier functions in non-centrosymmetric honeycomb lattices. ( a ) Crystal structure of a typical heteronuclear honeycomb lattice. Each unit cell, identified by two lattice vectors a 1 and a 2 , includes two inequivalent lattice sites, occupied by a cation-like and an anion-like atom, respectively. In sp materials, the upper valence bands can be mapped into four doubly degenerate Wannier functions centred around the anion. When the parent crystal is functionalized with hydrogen in a chair configuration the effect is twofold: (i) the effective ionic charge at each lattice site is increased by one unit and (ii) an additional Wannier function has to be included to accommodate the extra electrons. As shown in b , the in-plane projection of the corresponding centre is on top of the cation, while the other four Wannier functions remain localized around the anion, as in panel a . ( c ) Wannier function centres for group VI transition metal dichalcogenides (for example, MoS 2 , WSe 2 and so on). Six doubly degenerate Wannier functions are located around the chalcogens, while another one is located in the middle of the hexagonal cell. ( d ) Isosurface plot for the latter Wannier function in MoS 2 (Mo atoms in black and S atoms in yellow). Full size image Here, Z α and τ α are the charges and positions of the N ions in the unit cell and N el is the number of electrons. Let us first consider heteroatomic honeycomb lattices in which the electronic properties are determined by s and p orbitals, such as BN (monolayer SiC and ZnO, if realized, would also belong to this class). In Fig. 2a , we show the Wannier function centres of such systems, and by using equation (3) it is easy to show that the bulk formal polarization can be non-zero (see also Supplementary Table 1 ). A finite polarization charge thus appears at the edges of a nanoribbon made out of one of these honeycomb crystals, provided that the edge is not parallel to P (ref. 15 ). We have verified that indeed the polarization charge vanishes for armchair nanoribbons while it is maximal for perfect zigzag nanoribbons. Looking at, for example, the ideal case of zigzag edges, the polarization-induced electric field shifts the energy bands of the ribbon linearly in space, reducing the effective gap of the system. By increasing the width of the nanoribbon, a metal–insulator transition occurs as the top of the valence band reaches in energy the bottom of the conduction band. As shown in Fig. 1a , free carriers localize close to the edges of the nanoribbon with different character (electron or hole) on opposite sides. The density of free carriers at each edge increases with the width of the nanoribbon and, asymptotically, perfectly screens the polarization charge in agreement with equation (1). It is thus possible to tune such nanoribbons from a regime of small widths (few nanometres) in which there is a sizable electric field and negligible density of free carriers to an opposite regime for large widths (tens of nanometres or more) of vanishing electric fields but high metallicity. Metallicity of heteroatomic zigzag nanoribbons has been investigated theoretically in recent years [25] , [26] , [27] , and it has been pointed out that such 1D metallic channels can undergo magnetic transitions and eventually become half-metallic. However, no connection with the intrinsic polarization of the parent materials and with the existence of finite electric fields [28] has been drawn yet. As we shall discuss later, this is actually one of the key features that make some of these systems very promising for solar-energy applications. It is important to mention that depending on the edge termination, additional charges might appear at the boundaries. For instance, by terminating edge bonds with hydrogen, an additional ± e charge per unit length is introduced at opposite edges. Therefore, any specific termination does not neutralize the total charge at the edge, as termination effects can change it only by an integer number of electrons per unit length, while the polarization charge is typically a non-integer fraction of an electron per unit length. The only relevant exceptions are pristine III–V ribbons (that is, exactly BN) for which m =0, so that termination-induced charges might completely screen polarization effects. On the other hand, functionalized BN ribbons, discussed later, would be resilient against such mechanism. In addition, even in the case with m =0, by applying strain it would be possible to tune the polarization charge while leaving unaffected the termination effects, thus restoring a finite electric field (see also the Supplementary Note 1 for a detailed description of termination effects). From an experimental point of view, the main challenge would be to control the edge structure and chemistry. On the other hand, recent progress [29] , [30] , [31] in atomistic control over the edge structure of graphene nanoribbons has been quite spectacular and could be foreseeably extended to other honeycomb crystals. Nanoribbons of transition metal dichalcogenides In addition to sp materials, other honeycomb lattices can support a finite bulk polarization, starting from transition metal dichalcogenides (MX 2 ). Although these materials have been extensively studied in the last few years [32] , [33] , their bulk formal polarization has not been discussed so far. In such systems, one sublattice is occupied by a transition metal M while the other hosts two chalcogens X displaced in the vertical direction on opposite sides with respect to the plane of M atoms. In Fig. 2c , we show the Wannier function centres for the top seven valence bands when the transition metal belongs to group VI (M=Mo, W). Six centres lie close to the S atoms, which play the role of ‘anions’ (see also Supplementary Note 2 ), while the last one is located at the centre of the hexagonal cell and is associated with the Wannier function displayed in Fig. 2d . As a consequence, group VI transition metal dichalcogenides such as MoS 2 have a non-trivial (that is, m ≠0) formal polarization and their nanoribbons support a polar discontinuity, in exact analogy with what happens for sp materials. In addition, we mention that a polar discontinuity occurs also across inversion domain boundaries [34] , [35] , [36] that lie along zigzag directions and separate crystallites with opposite polarizations. Thus, transition metal dichalcogenides offer a broad choice in materials, chemistry and electronic structure, and represent one of the most promising experimental avenues to pursue. Indeed, polarization effects might be at the origin of metallic states already observed at inversion domain boundaries in MoSe 2 (ref. 36 ) and at the edge of MoS 2 nanoclusters [37] . Selective functionalization As a second different route to engineer polar discontinuities we suggest covalent atomic functionalizations, such as those with hydrogen or fluorine. We assume full coverage and we consider for simplicity a chair conformation, corresponding to functionalizations in alternating positions above and below the plane of the parent honeycomb lattice (see Supplementary Note 3 for a discussion on the different conformations of functionalized BN and their thermodynamic stability). In Fig. 2b , we show the Wannier function centres for a typical functionalized honeycomb lattice. We report results only for the case of hydrogen, as the case of fluorine is completely analogous. It is easy to verify that these covalent functionalizations change the value of m in equation (2) by one unit with respect to the parent material. As a consequence, we first note that functionalized nanoribbons would still support a polar discontinuity at the edges (and in particular III–V materials become less sensitive to termination-induced charges as m changes from 0 to 1, see Supplementary Table 1 ). Second, selective functionalization of a parent honeycomb lattice would create an interface between pristine and functionalized regions, introducing a polar discontinuity in the system. This situation is depicted in Fig. 1b , where we consider perfect zigzag interfaces (i.e., those giving rise to the largest polar discontinuity) between alternating stripes of pure and hydrogenated BN, similar to what happens in graphene ‘nanoroads’ [38] . As expected, free carriers localize at opposite interfaces. This case will be discussed at length in the last part of the paper, but we point out that the two regions (pristine and functionalized) remain obviously aligned with respect to each other and are close to a perfect lattice match (for example, for BN: a BN =2.51 Å and ). The experimental challenge is thus shifted to the selective functionalization of the parent crystal. To achieve this result, it is likely to be that techniques adopted for the functionalization of graphene [39] , [40] could be generalized to heteroatomic honeycomb crystals. Indeed, full coverage, double-sided hydrogenation of graphene (that is, graphane) has been realized in suspended samples by exposure to low-temperature hydrogen plasmas [41] . As far as fluorographene is concerned, a 1:1 carbon to fluorine ratio is achievable by functionalization with atomic fluorine formed by decomposition of xenon difluoride [42] , [43] . By combining this technique with scanning probe lithography, a pristine graphene nanoribbon has been isolated within a matrix of partially fluorinated graphene [44] . In addition, encouraging results have been already reported on the partial fluorination of BN nanotubes [45] and nanosheets [46] . Functionalized graphene/BN interfaces In view of the well-established experimental technology in growing single-layer graphene and BN, and the recent achievements [18] , [19] , [20] , [21] , [22] in obtaining sharp graphene/BN lateral heterostructures, it is of great interest to exploit these materials to engineer a polar discontinuity. Although pristine graphene is not an insulator and does not support a bulk polarization, its functionalized forms (graphane [41] and fluoro-graphene [42] , [43] ) are insulators and their formal polarization is constrained by symmetry to be zero [12] , [13] . Moreover, we have seen above that functionalized BN acquires a non-trivial bulk polarization ( m =1). Thus, full functionalization of existing planar graphene/BN heterostructures [18] , [19] , [20] , [21] , [22] will lead to the emergence of a polar discontinuity and a finite density of free carriers at the interfaces, as shown in Fig. 1c (we stress that this mechanism is completely different from the one that leads to metallicity in unfunctionalized graphene/BN interfaces [47] ). In addition, the intrinsic preference of these interfaces to grow along a zigzag direction [18] , [21] provides the optimal orientation to maximize the polar discontinuitiy. Functionalized nanotubes Although this paper is mainly devoted to 2D systems, we would like to illustrate what happens when these honeycomb lattices are rolled up in nanotubes and a finite polarization along the axis arises depending on the chirality of the nanotube [48] . Focusing on zigzag nanotubes, by selective functionalization one can introduce a polar discontinuity along the tube, as illustrated in Fig. 1d . Similar to what happens in 2D, a finite polarization charge builds up at the interfaces, creating an electric field that induces a charge reconstruction, with the appearance of electron- and hole-rich quantum dots. The charge density localized in these quantum dots is shown in Fig. 1d in the case of a (8,0) BN nanotube with selective hydrogen functionalization. The reduced dimensionality suggests that the effects of Coulomb interactions might be relevant for the electronic-structure properties of such quantum dots, similar to what happens in carbon-nanotube quantum dots [49] . The interaction-driven phenomena that might arise would then be interesting both from a fundamental and practical point of view, with particular emphasis towards quantum information applications [50] . In addition, even in the regime of small system sizes (when no charge is transferred in the quantum dots), the magnitude of the electric field in each segment might be easily tuned by varying the diameter of the nanotube and the distance between the interfaces. As we shall discuss in the following, this has significant consequences in solar-energy applications. First-principles simulations To support the general arguments presented above, we now use detailed, large-scale first-principles simulations to investigate a paradigmatic case study. For definiteness, we focus on selective hydrogen functionalization of BN (that we label as BNH 2 ), even though qualitatively similar results can be obtained using different parent materials and functional atoms, or any of the alternative approaches discussed above (and summarized in Table 1 ). Table 1 Methods and materials to engineer polar discontinuities. Full size table We simulate interfaces between pristine and functionalized BN within periodic boundary conditions, considering superlattices obtained by alternating BN and BNH 2 regions. As a consequence, two opposite interfaces are present within a simulation supercell, which is identified by two primitive lattice vectors. The first one defines the periodicity along the interface and can be determined by specifying the number of zigzag and armchair sections present, as shown in Fig. 3b : ( and p are positive coprime integers while a Z = a 2 and a A = a 1 +2 a 2 are translation vectors along the zigzag and armchair direction, respectively). The second lattice vector s 2 =2 q a 1 defines the periodicity of the superlattice in terms of the number of unit-cell repetitions q that define the width of each region. It is important to mention that the lattice vector s 1 alone is not sufficient to uniquely define the interface, as one still needs to specify the shape of the boundary (that is, which lattice sites should be assigned to each side of the interface). For simplicity we consider only interfaces that minimize the number of boundary atoms and bonds [51] . Different choices would affect only quantitatively the results, through the appearance of additional bound charges at the interface. 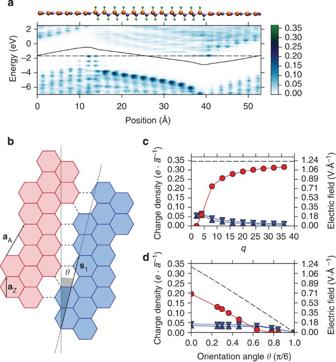Figure 3: Numerical results for BN–BNH2interfaces. (a) Planar average of the local density of states as a function of energy and position along an axis orthogonal to the interfaces, for aq=12 BN–BNH2superlattice withp=0 (zigzag interface), shown on top. The dashed line marks the Fermi energy, while the solid line denotes the planar average of the electrostatic potential energy. (b) Schematic representation of an arbitrary interface orientation. The lattice vector along the interface,, forms an angleθwith a zigzag direction;andp=1 here. (c) Free charge density (red circles, left axis) at each zigzag interface as a function of superlattice periodicity, expressed in units of, whereis the equilibrium lattice constant along the interface. The dashed line shows the asymptotic value given by equation (1), and up (down) blue triangles denote the residual average electric fields (right axis) inside BN (BNH2). (d) Same as incbut as a function of the interface orientation angleθfor aq=7 superlattice. The dashed line shows instead the free charge density in the limitq→∞ given by equation (5). Incandd, the scales of the left and right axes map charge densities and electric fields exactly into each other, so that, for example, a density read on the left axis will give the corresponding field on the right axis. Figure 3: Numerical results for BN–BNH 2 interfaces. ( a ) Planar average of the local density of states as a function of energy and position along an axis orthogonal to the interfaces, for a q =12 BN–BNH 2 superlattice with p =0 (zigzag interface), shown on top. The dashed line marks the Fermi energy, while the solid line denotes the planar average of the electrostatic potential energy. ( b ) Schematic representation of an arbitrary interface orientation. The lattice vector along the interface, , forms an angle θ with a zigzag direction; and p =1 here. ( c ) Free charge density (red circles, left axis) at each zigzag interface as a function of superlattice periodicity, expressed in units of , where is the equilibrium lattice constant along the interface. The dashed line shows the asymptotic value given by equation (1), and up (down) blue triangles denote the residual average electric fields (right axis) inside BN (BNH 2 ). ( d ) Same as in c but as a function of the interface orientation angle θ for a q =7 superlattice. The dashed line shows instead the free charge density in the limit q →∞ given by equation (5). In c and d , the scales of the left and right axes map charge densities and electric fields exactly into each other, so that, for example, a density read on the left axis will give the corresponding field on the right axis. Full size image We first focus on the case of a perfect zigzag interface ( p =0), when we have a finite polarization charge density with opposite signs at each interface. These polarization charges create an electric field inside both BN and BNH 2 , as can be clearly seen in Fig. 3a examining the finite slope of the macroscopic and planar average [52] of the electrostatic potential energy (solid line). In Fig. 3 , we also show the average local density of states as a function of energy and position along the direction orthogonal to the interfaces. As a consequence of the electric field, the electronic bands shift linearly as a function of position. For sufficiently large widths (as in Fig. 3a ), this leads to an energy overlap between the conduction and valence bands of the two interfaces, and to a charge redistribution with the creation of electron and hole pockets [10] , [14] . The Fermi energy (dashed line) intersects both the top of the valence band and the bottom of the conduction band so that the system has become metallic, as expected. Figure 1b shows the excess charge density obtained by integrating the local density of states to take into account the partial depletion of the valence bands (for holes) and the filling of the conduction bands (for electrons). Both figures make it clear that excess electrons and holes are separated in space and reside on opposite interfaces, partially screening the polarization charges. In Fig. 3c , we report the density of free carriers for different widths of the ribbons (red circles). As the periodicity of the superlattice increases, the charge of free electrons and holes also increases as a result of a larger overlap between conduction and valence bands. As the free charge has an opposite sign with respect to the polarization charge, the overall charge density at each interface decreases together with the electric field in both materials (blue triangles in Fig. 3c ). Asymptotically, the free charge completely balances the polarization charge according to equation (1) and the electric fields vanish, thus preventing a polar catastrophe [8] . Indeed, in Fig. 3c the density of free carriers approaches asymptotically the polarization charge obtained from the bulk formal polarizations of BN and BNH 2 (black dashed line). If the two materials were perfectly lattice-matched, we would have, from the discussion on Wannier functions above (equations (1) and (2)), |λ P |= e /(3 a ). Owing to the piezoelectric properties of these materials, λ P is slightly larger than as a result of the finite strain necessary to reach a common equilibrium lattice constant along the interface [14] . Let us now consider an arbitrary interface orientation that can be identified by the angle θ between the lattice vector along the interface, s 1 , and the pure zigzag direction, a Z , so that According to equations (1) and (2), the polarization charge density gradually decreases down to zero as θ goes from zero (pure zigzag, p =0) to π /6 (pure armchair, ). In particular, neglecting for simplicity piezoelectric effects, we find Thus, we expect that the appearance of finite electric fields and the presence of a metal–insulator transition are not restricted to the case θ =0, although their effects are depressed as we approach θ = π /6. Figure 3d shows the free charge density and the electric fields in BN and BNH 2 for several values of θ corresponding to different combinations of and p . All simulations have been performed keeping fixed the periodicity of the superlattice ( q =7). Despite the small width of the system, the free charge density survives over a wide range of angles, thus suggesting robustness with respect to the interface orientation. In addition, by incrementing the periodicity of the superlattice, the free charge density could be further increased and asymptotically reach the dashed line representing the polarization charge in equation (5), as it happens in the θ =0 case shown in Fig. 3c . We have presented different approaches to obtain polar discontinuities in honeycomb lattices, supporting these predictions with first-principles simulations. First, we highlight that a finite-width nanoribbon introduces a polar discontinuity with vacuum if the parent material supports a finite formal polarization. This happens for heteroatomic honeycomb crystals such as BN and its functionalized derivatives, and for transition metal dichalcogenides, such as molybdenum disulfide. The existence of a polar discontinuity at the edges elucidates why metallicity can arise in honeycomb nanoribbons [25] , [26] , [27] or at inversion domain boundaries [36] . Second, we show that covalent atomic functionalizations, for example, with hydrogen or fluorine, can change the bulk polarization of a honeycomb lattice. Thus, covalent functionalizations can be used to engineer polar discontinuities in 2D materials or 1D nanotubes simply by introducing interfaces between functionalized and pristine sections. In addition, as covalent functionalizations open a gap in graphene, they can be exploited to engineer polar discontinuities in existing graphene/BN interfaces [18] , [19] , [20] , [21] , [22] , without the need for selective functionalization. We believe that engineering polar discontinuities in honeycomb lattices will provide a novel platform for manifold applications. First, 1D channels of free carriers along the interfaces could be exploited for circuitry in new-generation ultra-thin and flexible electronics. Indeed, current signals between different units of a device could be transmitted along such 1D channels, surrounded by insulating bulk materials, exceeding the limits of lithography in current electronic devices. Moreover, the reduced dimensionality of the channels gives rise to magnetic instabilities [14] that could be useful in spintronics applications. Second, and even more compelling, we envision a fruitful employment in solar-energy technology for the realization of light-harvesting devices. Indeed, the ‘bulk’ interior of these systems is insulating and is an active region where photons can be absorbed, creating electron–hole pairs. For narrow systems, the polarization charges at the interfaces or edges are not compensated and thus naturally create an electric field (we note in passing that this is different from what has been done in recent photovoltaic devices based on transition metal dichalcogenides [53] , [54] , [55] , [56] , where metallic gates have been employed to create a p – n junction). Once the electron–hole pair is created, the electric field separates the electron and the hole, and guides them towards opposite interfaces, where the 1D wires naturally collect and transport them. In addition, the electric field shifts in space the conduction and valence band extrema, and creates a variable effective gap depending on the spatial extension of the exciton, with an ensuing tunability of the cell efficiency. Furthermore, several systems with different widths and materials composition could be integrated into a single device to optimize the range of photon frequencies that can be absorbed. First-principles simulations All first-principles calculations reported here are carried out within density-functional theory by using the PWscf code of the Quantum-ESPRESSO distribution [57] with the Perdew–Burke–Ernzerhof exchange-correlation functional [58] . An ultrasoft pseudopotential description [59] of the ion–electron interactions is adopted. Energy cutoffs are set to 60 and 300 Ry, respectively, for the electronic wavefunctions and the charge density in the case of BN/BNH 2 superlattices. For zigzag interfaces, a 1 × 6 × 1 shifted Monkhorst–Pack grid is used to sample the Brillouin zone together with a 0.01-Ry Marzari–Vanderbilt smearing [60] . To simulate a 2D system irrespective of the three-dimensional periodicity requirements of plane-wave basis sets, a vacuum layer of 20 Å is added between periodic replicas in the vertical direction. Relaxed structures are obtained within the Broyden–Fletcher–Goldfarb–Shanno method by requiring that the forces acting on atoms are below 0.026 eV Å −1 and the residual stress on the cell is <0.5 kbar. Some simulations have been performed without relaxation to simplify the calculations without qualitatively affecting our results. We notice that the well-known density-functional theory limitations in predicting energy gaps influence only quantitatively the relation between free charge density, electric fields and width of the system, without changing the general physical picture or its asymptotic limits. Maximally localized Wannier functions have been computed using the Wannier90 code (ref. 61 ). How to cite this article: Gibertini, M. et al . Engineering polar discontinuities in honeycomb lattices. Nat. Commun. 5:5157 doi: 10.1038/ncomms6157 (2014).